A versatilecis-acting inverter module for synthetic translational switches Artificial genetic switches have been designed and tuned individually in living cells. A method to directly invert an existing OFF switch to an ON switch should be highly convenient to construct complex circuits from well-characterized modules, but developing such a technique has remained a challenge. Here we present a cis -acting RNA module to invert the function of a synthetic translational OFF switch to an ON switch in mammalian cells. This inversion maintains the property of the parental switch in response to a particular input signal. In addition, we demonstrate simultaneous and specific expression control of both the OFF and ON switches. The module fits the criteria of universality and expands the versatility of mRNA-based information processing systems developed for artificially controlling mammalian cellular behaviour. Artificial genetic circuits have been constructed on the basis of logical topology by employing cis- and trans -regulatory modules [1] . The introduction of designed circuits to intracellular environments has real-world applications in fields relevant to human health, the production of materials and energy and the environment [2] . The central process in many genetic circuit applications is the detection of a signal molecule that represents a particular cellular state, followed by the transmission of that signal to the circuit. Many genetic circuits have been constructed by employing transcriptional regulatory proteins under the control of a signalling input molecule [3] . In a newly developed approach, an RNA molecule functions as a central processor that regulates gene expression under the control of an input signal: an ON switch activates the expression of an output gene, whereas an OFF switch represses it [4] , [5] , [6] . Switches have been constructed on the basis of a variety of molecular design principles. For example, a designed mRNA switch composed of an RNA aptamer [7] for a specific molecule, and an open reading frame (ORF) of interest will regulate translation depending on the interaction between the aptamer and its ligand [8] , [9] , [10] , [11] , [12] , [13] , [14] . In previous reports, the RNA devices for OFF and ON switches have had to be designed and tuned individually. For example, ribozyme-based ON and OFF switches have been designed and constructed by fusing an RNA aptamer to a hammerhead ribozyme [9] . The aptamer regulates the activity of the ribozyme depending on the presence or absence of its ligand. However, the fused components of each switch have to be tuned and screened individually to optimize the performance of the switch. In an alternative approach, a trans -acting effector and sensor pair was employed to achieve an inversion between the OFF and ON switches. In this system, two linked OFF switches function together as an ON switch: the first switch outputs a repressor protein that acts as an input signal for the second switch. However, this approach requires multiple trans -acting modules to invert the switches, and a shortage of well-characterized modules is a crucial problem in the field. The use of a set of modules also risks disturbing intrinsic networks, unless the modules are confirmed to not interact with these networks. Thus, it would be highly advantageous to develop a versatile method to invert an OFF switch to an ON switch in cis with corresponding performance. In this study, we develop a cis -acting switch inverter. Insertion of the cis -acting module into a target mRNA sequence inverts an OFF switch to an ON switch that responds to the same input molecule with a similar sensitivity and reactivity. For this purpose, we employ a protein-responsive OFF switch set within an mRNA Molecule [10] , [15] . This switch binds to an input protein at a specific site in the 5′-untranslated region (UTR) to block translation. As expected, derived ON switches respond to the input consistently with their parental OFF switches. The application of this inserted element to directly invert a switch would increase the modularity and versatility of RNA-based synthetic devices. Symmetrically controlling two switches with the same input molecule would allow us to construct genetic circuits with a smaller number of molecular parts. Design of the cis -acting module to invert OFF switches In the OFF switch ( Fig. 1a ), a protein serves as an input that binds to a natural or an artificial RNA aptamer to repress translation. We inverted the OFF switch to an ON switch using a cis -regulatory module ( Supplementary Fig. S1 ) based on a translation-dependent translation repression mechanism. To construct a switch-inverting component, we exploited the phenomenon of nonsense-mediated mRNA decay (NMD) [16] , which is a well-known quality-control system for mRNAs in eukaryotic cells. During NMD, mRNAs containing nonsense mutations are degraded to prevent the expression of truncated or erroneous proteins. In mammalian systems, a premature termination codon (PTC) located upstream of a splice site is recognized as a nonsense mutation, thus promoting degradation. We prepared a synthetic mRNA that contains a bait ORF and tandem PTCs, followed by a β-globin intron and an internal ribosome entry site (IRES) ( Fig. 1b ). The tandem PTCs of the bait ORF were positioned more than 500 nucleotides upstream of the splice site to effectively trigger NMD [17] . Insertion of the component into a site between a sensory RNA aptamer motif that binds to the input molecules and the first codon of the output protein should invert an OFF switch to an ON switch that is responsive to the same input molecule. In the absence of the input signal, translational termination of the bait ORF triggers degradation of the mRNA and essentially eliminates the IRES-driven protein output from the destabilized mRNA ( Fig. 1c ). However, in the presence of the input signal, translation of the bait ORF should be blocked in the same manner as in the original OFF switch so that the IRES can drive the synthesis of the output protein from the stabilized ON switch mRNA ( Fig. 1d ). 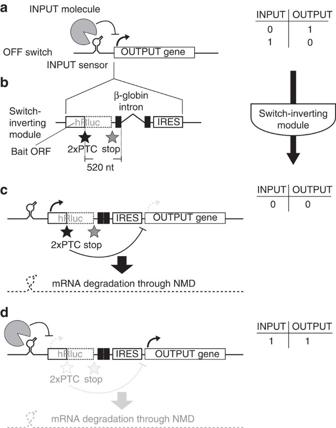Figure 1: Design of the switch-inverting module. (a) Construction of an OFF switch mRNA sequence. An RNA sensory motif that binds to an input molecule is inserted into the 5′-UTR of an mRNA sequence encoding an output gene. The binding of the input molecule to the mRNA inhibits the expression of the output (input=1, output=0), which does not occur in the absence of the input molecule (input=0, output=1). (b) Switch-inverting module for the OFF switch mRNA sequence. The module consists of a bait ORF (N-terminal 152 amino acids ofRenillaluciferase) followed by an intron and an IRES. The two PTCs (2 × PTCs) of the bait ORF are located more than 500 nucleotides (nt) upstream of the splice site of the intron to enhance the efficiency of mRNA degradation. The module should be inserted between the RNA motif and the first codon of the OFF switch to generate the ON switch. (c) Behaviour of the inverted ON switch in the absence of the target molecule (input=0). The termination of the translation of the bait ORF triggers mRNA degradation, and the output gene is not sufficiently expressed from the destabilized mRNA (output=0). (d) Behaviour of the ON switch in the presence of the input (input=1). The translation of the bait ORF is blocked in the same manner as in the original OFF switch, and mRNA degradation is therefore not triggered. As a result, the IRES-driven output protein is stably synthesized from the ON switch (output=1). Figure 1: Design of the switch-inverting module. ( a ) Construction of an OFF switch mRNA sequence. An RNA sensory motif that binds to an input molecule is inserted into the 5′-UTR of an mRNA sequence encoding an output gene. The binding of the input molecule to the mRNA inhibits the expression of the output (input=1, output=0), which does not occur in the absence of the input molecule (input=0, output=1). ( b ) Switch-inverting module for the OFF switch mRNA sequence. The module consists of a bait ORF (N-terminal 152 amino acids of Renilla luciferase) followed by an intron and an IRES. The two PTCs (2 × PTCs) of the bait ORF are located more than 500 nucleotides (nt) upstream of the splice site of the intron to enhance the efficiency of mRNA degradation. The module should be inserted between the RNA motif and the first codon of the OFF switch to generate the ON switch. ( c ) Behaviour of the inverted ON switch in the absence of the target molecule (input=0). The termination of the translation of the bait ORF triggers mRNA degradation, and the output gene is not sufficiently expressed from the destabilized mRNA (output=0). ( d ) Behaviour of the ON switch in the presence of the input (input=1). The translation of the bait ORF is blocked in the same manner as in the original OFF switch, and mRNA degradation is therefore not triggered. As a result, the IRES-driven output protein is stably synthesized from the ON switch (output=1). Full size image Derivation of ON switches from OFF switches We inserted this module into a previously developed protein-responsive OFF switch mRNA sequence (OFF-Kt) containing the sequence of the enhanced green fluorescent protein (EGFP) gene as an output and the RNA motif (K-turn, referred to as Kt) that detects archaeal ribosomal protein L7Ae as an input [10] . Thus, the inverted ON switch mRNA (ON-Kt) should detect L7Ae and activate the expression of EGFP ( Fig. 2a ). The constructed plasmid was transfected into HeLa cells together with an input plasmid expressing either L7Ae or the MS2 coat protein as a cognate or noncognate protein, respectively. DsRed-Express translated from the IRES of the input plasmid was used as an indicator for the input ( Fig. 2a–e ). Fluorescence microscopy analysis demonstrated that effective expression of EGFP from ON-Kt occurred in the presence of L7Ae ( Fig. 2c ), whereas effective EGFP expression was not observed, even 24 h after transfection of the plasmid carrying the MS2 coat protein ( Fig. 2b ). When Kt was replaced with a defective Kt (ON-dKt) that cannot bind L7Ae, EGFP was not synthesized effectively, regardless of cognate protein expression ( Fig. 2e ), demonstrating that the expression of L7Ae did not affect NMD or the IRES. Flow-cytometry analysis revealed that cells transfected with the cognate pair of plasmids (L7Ae/ON-Kt) showed five- to sevenfold higher levels of EGFP fluorescence in average than those with noncognate pairs ( Fig. 2f ). These results indicate that the insertion of the cis -acting module into the mRNA effectively inverted the OFF switch to the ON switch. 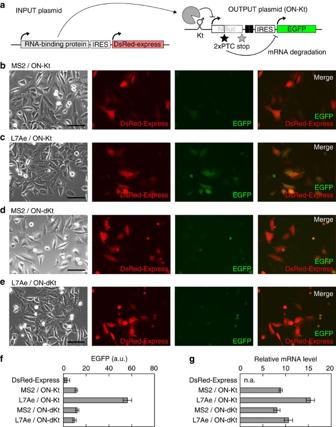Figure 2: Behaviour of an inverted ON switch generated via insertion of the module into an OFF switch. (a) Construction of the INPUT and OUTPUT plasmids transfected into HeLa cells in this study. The INPUT plasmids express either L7Ae or the MS2 coat protein (MS2) as a cognate or noncognate RNA-binding protein, respectively. DsRed-Express is also synthesized from the INPUT plasmid, driven by the IRES. An OUTPUT plasmid expresses ON-switch mRNAs containing K-turn (Kt) or defective K-turn (dKt) as either an active or defective sensory motif, respectively. EGFP driven by the IRES is synthesized from the OUTPUT plasmid. (b–e) Images of cells captured via fluorescence microscopy. DsRed-Express synthesized together with L7Ae (c,e) or MS2 (b,d) is shown in red. EGFP outputs from an ON switch with either an active (b,c; ON-Kt) or a defective (d,e; ON-dKt) sensor are shown in green. These two fluorescent signals are merged and shown in the right most pictures. Scale bars, 200 μm. (f) The mean intensity of EGFP fluorescence of transfected cells. HeLa cells shown inb–ewere analysed using a flow cytometer, FACSAria. Cells expressing only DsRed-Express were used as the negative control (DsRed-Express). Bars and error bars represent the mean and s.d., respectively, of three triplicate experiments (n=9). (g) The levels of ON-switch mRNAs, as determined by quantitative RT–PCR. To eliminate the noise from untransfected cells, the results are normalized by employing the mRNA of neomycin-resistant gene transcribed from the OUTPUT plasmid in cells. Bars and error bars represent the mean and s.d., respectively, of three triplicate experiments (n=9). n.a., not analysed. All experiments inb–gwere carried out 24 h after the transfection of 100 ng of the indicated OUTPUT plasmid and 20 ng of the INPUT plasmid together with 480 ng of the noncognate INPUT plasmid. Figure 2: Behaviour of an inverted ON switch generated via insertion of the module into an OFF switch. ( a ) Construction of the INPUT and OUTPUT plasmids transfected into HeLa cells in this study. The INPUT plasmids express either L7Ae or the MS2 coat protein (MS2) as a cognate or noncognate RNA-binding protein, respectively. DsRed-Express is also synthesized from the INPUT plasmid, driven by the IRES. An OUTPUT plasmid expresses ON-switch mRNAs containing K-turn (Kt) or defective K-turn (dKt) as either an active or defective sensory motif, respectively. EGFP driven by the IRES is synthesized from the OUTPUT plasmid. ( b – e ) Images of cells captured via fluorescence microscopy. DsRed-Express synthesized together with L7Ae ( c , e ) or MS2 ( b , d ) is shown in red. EGFP outputs from an ON switch with either an active ( b , c ; ON-Kt) or a defective ( d , e ; ON-dKt) sensor are shown in green. These two fluorescent signals are merged and shown in the right most pictures. Scale bars, 200 μm. ( f ) The mean intensity of EGFP fluorescence of transfected cells. HeLa cells shown in b – e were analysed using a flow cytometer, FACSAria. Cells expressing only DsRed-Express were used as the negative control (DsRed-Express). Bars and error bars represent the mean and s.d., respectively, of three triplicate experiments ( n =9). ( g ) The levels of ON-switch mRNAs, as determined by quantitative RT–PCR. To eliminate the noise from untransfected cells, the results are normalized by employing the mRNA of neomycin-resistant gene transcribed from the OUTPUT plasmid in cells. Bars and error bars represent the mean and s.d., respectively, of three triplicate experiments ( n =9). n.a., not analysed. All experiments in b – g were carried out 24 h after the transfection of 100 ng of the indicated OUTPUT plasmid and 20 ng of the INPUT plasmid together with 480 ng of the noncognate INPUT plasmid. Full size image This switch-inverting component was designed based on the concept that the switch mRNAs are degraded in a translation-dependent manner, whereas they are protected from degradation in the presence of the cognate input. The amount of switch mRNA present 24 h after transfection was determined via quantitative reverse transcription PCR (RT–PCR) analysis ( Fig. 2g ). As expected, the amount of ON switch mRNA in cells transfected with the cognate pairs (L7Ae/ON-Kt) was 1.7-fold higher than in cells with noncognate pairs, showing that the inserted module increased the steady-state levels of the switch mRNA in the cells. This result is consistent with the findings of a previous study demonstrating that blocking translation initiation rescued the level of nonsense-containing mRNA with a similar efficiency [18] . Switch-inversion based on NMD To further investigate the molecular mechanism of the designed module, we constructed a defective module, in which the tandem PTCs were removed, resulting in 43 nucleotides in length between the stop codon of the bait ORF and the splice site of the intron (referred to as ONn; Fig. 3a ). We inserted ONn to the parental OFF switch and found that removal of PTCs increased EGFP production even in the absence of L7Ae, and therefore disrupted the ability of the inverter module ( Fig. 3a , see also Supplementary Fig. S2 for comparison of the results from different cytometers). This suggests that basal repression of our module depends on PTCs. 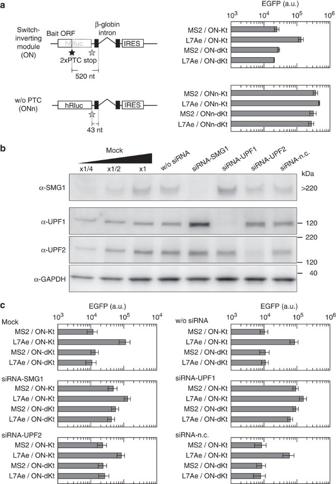Figure 3: Dependency of inverted switches on PTC and NMD factors. (a) A switch-inverting module without PTC (ONn). Schematic illustrations of the modules and EGFP fluorescence from switches inverted by the modules are shown in left and right, respectively. The level of EGFP was determined using a flow cytometer, BD Accuri (see alsoSupplementary Fig. S2), 24 h after transfection of 100 ng of the indicated OUTPUT plasmid with 20 ng of cognate and 480 ng of noncognate INPUT plasmids. Bars and error bars represent the mean and s.d., respectively, of three replicates. (b) siRNA-induced knockdown of NMD factors: SMG1, UPF1 and UPF2. siRNAs to SMG1, UPF1, UPF2 or a non-silencing negative control siRNA (siRNA-n.c.) were transfected into HeLa cells. Forty-eight hours after the transfection, total protein was extracted and subjected to western blotting analysis. Glyceraldehyde 3-phosphate dehydrogenase (GAPDH) was also analysed as an internal control of the lysates. w/o siRNA indicates cells treated with only transfection reagent. The left three lanes were twofold serial dilutions of the lysate from untreated HeLa cells (mock). (c) Behaviour of inverted switches in siRNA-treated cells. Forty-eight hours after the transfection of siRNAs, cells were transfected with the plasmids. Plasmid transfection and analytical procedure were the same as ina. Bars and error bars represent the mean and s.d., respectively, of three replicates. Inaandc, cells were transfected with 100 ng of the indicated OUTPUT plasmid with 20 ng of cognate and 480 ng of noncognate INPUT plasmids. Figure 3: Dependency of inverted switches on PTC and NMD factors. ( a ) A switch-inverting module without PTC (ONn). Schematic illustrations of the modules and EGFP fluorescence from switches inverted by the modules are shown in left and right, respectively. The level of EGFP was determined using a flow cytometer, BD Accuri (see also Supplementary Fig. S2 ), 24 h after transfection of 100 ng of the indicated OUTPUT plasmid with 20 ng of cognate and 480 ng of noncognate INPUT plasmids. Bars and error bars represent the mean and s.d., respectively, of three replicates. ( b ) siRNA-induced knockdown of NMD factors: SMG1, UPF1 and UPF2. siRNAs to SMG1, UPF1, UPF2 or a non-silencing negative control siRNA (siRNA-n.c.) were transfected into HeLa cells. Forty-eight hours after the transfection, total protein was extracted and subjected to western blotting analysis. Glyceraldehyde 3-phosphate dehydrogenase (GAPDH) was also analysed as an internal control of the lysates. w/o siRNA indicates cells treated with only transfection reagent. The left three lanes were twofold serial dilutions of the lysate from untreated HeLa cells (mock). ( c ) Behaviour of inverted switches in siRNA-treated cells. Forty-eight hours after the transfection of siRNAs, cells were transfected with the plasmids. Plasmid transfection and analytical procedure were the same as in a . Bars and error bars represent the mean and s.d., respectively, of three replicates. In a and c , cells were transfected with 100 ng of the indicated OUTPUT plasmid with 20 ng of cognate and 480 ng of noncognate INPUT plasmids. Full size image We next knocked down NMD regulatory protein factors (SMG1, UPF1 and UPF2) using short interfering RNAs (siRNAs) ( Fig. 3b ). Two days after the transfection of siRNAs, we transfected the same sets of plasmids and assessed the behaviour of the inverted switches. Knockdown of these factors increased EGFP expression and diminished further upregulation of EGFP expression in the absence and presence of L7Ae, respectively ( Fig. 3c ), indicating that inversion of the switch depends on these factors. In addition, we shortened the distance between PTCs and the spliced site of the module ( Supplementary Fig. S3 ). Shortening the distance to 320 nucleotides was sufficient for the module to invert the switch. However, distances shorter than this, such as 160 nucleotides proved insufficient in keeping with previous evidence that the shorter distances were less effective for triggering NMD [17] . Taken together, these results indicate that the function of our inverter module depends on the mechanism of NMD. Dose and affinity response of parental and inverted switches To investigate the performance of the switch-inverting module, we next assessed whether an inverted ON switch preserved the effectiveness of the input molecule compared with the parental OFF switch. We analysed the responses of the ON and OFF switches as a function of the level of input protein ( Fig. 4a , Supplementary Figs S4 and S5 ). We evaluated the behaviour of the switches by four different analytical procedures and found that the obtained values were very similar to each other (see Supplementary Fig. S6 and Methods for details of analytical procedure). As the amount of the transfected plasmid expressing L7Ae increased, the output EGFP fluorescence from the ON switch increased ( Fig. 4a and Supplementary Fig. S4 ; ON-Kt) in a pattern that was inversely related to that observed for the OFF switch ( Fig. 4a and Supplementary Fig. S4 ; OFF-Kt). For further validation, we employed an alternative binding pair: Bacillus ribosomal protein S15 and its corresponding RNA motif (Fr15) from 16S ribosomal RNA [19] ( Fig. 4a and Supplementary Fig. S5 ). The observed correlation between the behaviour of the parental OFF and inverted ON switches was similar to that of the L7Ae system ( Fig. 4a ; ON-Fr15 and OFF-Fr15, see also Supplementary Fig. S7 ). In addition, western blot analyses were performed to determine the input protein levels under the experimental conditions ( Fig. 4b,c ). We confirmed that expression level of L7Ae or S15 increases depending on the amounts of the input plasmid (0.2–5-fold to the output plasmid) and is not saturated under our experimental conditions. 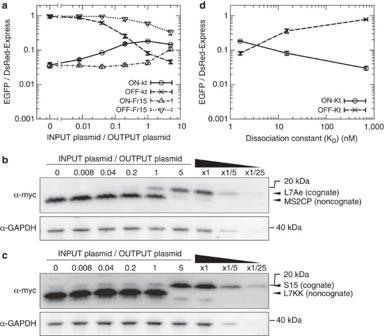Figure 4: Correlation of the sensitivity and reactivity between the inverted ON switches and parental OFF switches. (a) Behaviour of the switches as a function of the amount of input. Thexaxis shows the ratio of the INPUT plasmids expressing cognate RNA-binding proteins to the OUTPUT plasmids for the indicated switches (100 ng). The total plasmid content was adjusted up to 600 ng using noncognate plasmids. Twenty-four hours after transfection, individual cells were analysed using FACSAria. Geometrical mean values of the ratio between EGFP and DsRed-Express signals in a cell were shown. ON-Fr15 and OFF-Fr15 are switches responsive toBacillusribosomal protein S15 instead of L7Ae. Data points and error bars represent the mean and s.d., respectively, of three replicates. SeeSupplementary Fig. S4(ON-Kt and OFF-Kt) andSupplementary Fig. S5(ON-Fr15 and OFF-Fr15) for plots produced from this analysis. (b,c) Western blotting analysis of input proteins is shown. Total protein from the transfected cells shown inawas extracted 24 h after transfection and subjected to western blotting analysis. Cognate (L7Ae (b) and S15 (c)) and noncognate (MS2CP (b) and L7KK (c)) input proteins were detected using anti-myc antibody. Glyceraldehyde 3-phosphate dehydrogenase (GAPDH) was also analysed as an internal control of the lysates. The right three lanes were fivefold serial dilutions of the lysate prepared in the same condition as the ratio of INPUT plasmid/OUTPUT plasmid equal to 5. Representative result from the three independent experiments was shown. (d) Behaviour of the switches as a function of the affinity between the input protein and the corresponding sensory motif in the switch. SeeSupplementary Fig. S8for plots generated from this analysis. Figure 4: Correlation of the sensitivity and reactivity between the inverted ON switches and parental OFF switches. ( a ) Behaviour of the switches as a function of the amount of input. The x axis shows the ratio of the INPUT plasmids expressing cognate RNA-binding proteins to the OUTPUT plasmids for the indicated switches (100 ng). The total plasmid content was adjusted up to 600 ng using noncognate plasmids. Twenty-four hours after transfection, individual cells were analysed using FACSAria. Geometrical mean values of the ratio between EGFP and DsRed-Express signals in a cell were shown. ON-Fr15 and OFF-Fr15 are switches responsive to Bacillus ribosomal protein S15 instead of L7Ae. Data points and error bars represent the mean and s.d., respectively, of three replicates. See Supplementary Fig. S4 (ON-Kt and OFF-Kt) and Supplementary Fig. S5 (ON-Fr15 and OFF-Fr15) for plots produced from this analysis. ( b , c ) Western blotting analysis of input proteins is shown. Total protein from the transfected cells shown in a was extracted 24 h after transfection and subjected to western blotting analysis. Cognate (L7Ae ( b ) and S15 ( c )) and noncognate (MS2CP ( b ) and L7KK ( c )) input proteins were detected using anti-myc antibody. Glyceraldehyde 3-phosphate dehydrogenase (GAPDH) was also analysed as an internal control of the lysates. The right three lanes were fivefold serial dilutions of the lysate prepared in the same condition as the ratio of INPUT plasmid/OUTPUT plasmid equal to 5. Representative result from the three independent experiments was shown. ( d ) Behaviour of the switches as a function of the affinity between the input protein and the corresponding sensory motif in the switch. See Supplementary Fig. S8 for plots generated from this analysis. Full size image Next, we examined the behaviours of the parental and inverted switches in response to the affinity of the input ( Fig. 4d and Supplementary Fig. S8 ). We have previously reported that the K37A mutant (L7K) and the K37A, K78A double mutant (L7KK) derived from L7Ae bind Kt more weakly in vitro ; these mutants exhibit dissociation constants ( K D ) of 15 and 680 nM, respectively, in contrast to the 1.6 nM K D of L7Ae [20] . When L7Ae was replaced with these variants, the output EGFP expression from OFF-Kt increased as the K D value increased ( Fig. 4d ; OFF-Kt), whereas that from ON-Kt decreased in a symmetrical manner ( Fig. 4d ; ON-Kt). Taken together, these data indicate that the switch-inverting module can universally derive ON switches from parental OFF switches. The ON and OFF switches show similar efficiencies in responding to the same input in relation to the amount of the input molecule and the affinity of the interaction between the input and the sensory RNA motif. Ideally, the response of the inverted switch to the input signal should be exactly the opposite of the response of the parental switch. The dynamic range between the basal (repressed) and fully released state of the inverted ON-Fr15 switch was similar to that between the basal (released) and fully repressed state of the parental OFF-Fr15 switch ( Fig. 4a ). In contrast, the absolute output values corresponding to the repressed and released states of the two switches were different under the same conditions. If the absolute values after the conversion need to be adjusted for some applications, the mRNA levels in a cell can be optimized by altering the strength of the promoter or the efficiency of plasmid uptake; this procedure will likely compensate for the difference by vertically shifting the curves shown in Fig. 4a . In fact, dilution of the output plasmids altered the absolute values of EGFP expression but maintained similar dynamic range before and after the inversion, suggesting that NMD component was not saturated under the experimental conditions ( Supplementary Fig. S9 ). We also revealed that our module is effective under the control of alternative promoters such as Rous sarcoma virus promoter or elongation factor-1α promoter in addition to cytomegalovirus promoter ( Supplementary Fig. S10 ). These promoters altered the level of EGFP expression while maintaining a similar fold change before and after the inversion as in the case of plasmid dilution, indicating that output protein level from an inverted switch can be tuned by employing different promoters and/or the different concentration of the plasmids. The minimum and maximum limits of the output expression determine the usable range of the inverted switch. In the case of the L7Ae-responsive switches described above, the corresponding usable range was narrowed after the conversion of OFF-Kt into ON-Kt ( Fig. 4a ). The response of ON-Kt reached its maximal limit at an input protein level that only suppressed OFF-Kt to half of its maximal level (corresponding to more than a 10-fold difference), and this restricted limit could cause difficulties with regards to the range of use. The IRES-driven synthesis of the output protein is blocked after the IRES is degraded as a consequence of NMD. Therefore, very efficiently coupling NMD to IRES inactivation could reduce the minimum output level of the system and help to solve this problem. Enhancing the activity of the IRES could also improve the performance of the module by increasing the output level because IRES-driven protein synthesis is generally less effective than cap-dependent translation. Controlling a cellular phenotype and multiple genes We next investigated to see whether our system could control a cellular phenotype via the apoptosis pathways ( Fig. 5 ). We have shown that the OFF switch could repress translation of anti-apoptotic Bcl-xL to induce apoptosis [12] . Likewise, we designed an apoptosis-controllable switch in which the output EGFP protein was replaced with pro-apoptotic Bim-EL to express Bim-EL in the input-protein-, L7Ae, dependent manner ( Fig. 5a ). After the transfection of the corresponding plasmids, we evaluated the number of annexin V-positive apoptotic cells by using a flow cytometer. As expected, annexin V-positive cells were increased specifically when the cognate pair of the plasmids was injected (L7Ae and ON-Kt-B, Fig. 5b ). The efficiency of the induced apoptosis was consistent with the previous result [12] . 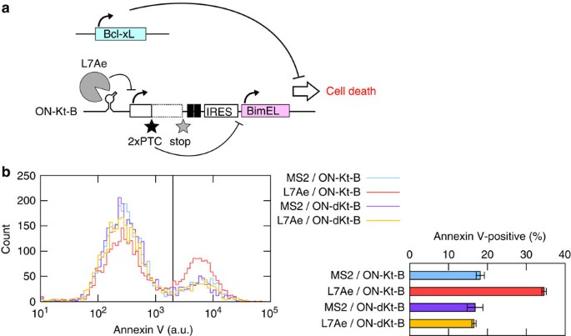Figure 5: Induction of cell death using an inverted switch. (a) Schematic illustration of the experiment. Together with the INPUT plasmids (500 ng), we transfected two plasmids: one expressing anti-apoptotic gene, Bcl-xL (10 ng) and ON-Kt-B (or dKt, 100 ng), which outputs apoptotic gene, Bim-EL instead of EGFP. (b) Induction of annexin V-positive cells. For transfection, 20 ng of cognate and 480 ng of noncognate INPUT plasmids were mixed. The left panel shows histograms of Pacific Blue-labelled anti-annexin V using FACSAria. A black line indicates a threshold used in this analysis. The right panel shows a ratio of annexin V-positive cells to the transfected cells. Bars and error bars represent the mean and s.d., respectively, of two replicates. Figure 5: Induction of cell death using an inverted switch. ( a ) Schematic illustration of the experiment. Together with the INPUT plasmids (500 ng), we transfected two plasmids: one expressing anti-apoptotic gene, Bcl-xL (10 ng) and ON-Kt-B (or dKt, 100 ng), which outputs apoptotic gene, Bim-EL instead of EGFP. ( b ) Induction of annexin V-positive cells. For transfection, 20 ng of cognate and 480 ng of noncognate INPUT plasmids were mixed. The left panel shows histograms of Pacific Blue-labelled anti-annexin V using FACSAria. A black line indicates a threshold used in this analysis. The right panel shows a ratio of annexin V-positive cells to the transfected cells. Bars and error bars represent the mean and s.d., respectively, of two replicates. Full size image Finally, we performed simultaneous regulation of two independent mRNAs by the OFF and ON switch ( Fig. 6 ). We analysed the behaviour of the inverted switches (ON-Kt or ON-dKt) and their modified parental switches (OFF-Kt or OFF-dKt) at the same time ( Fig. 6a ). As expected, both ON and OFF switches containing Kt were specifically up- and downregulated EGFP and enhanced cyan fluorescent protein as an output, respectively, in the presence of L7Ae. Notably, each OFF or ON switch incorporated into the same cell did not affect the function of its counterpart. Furthermore, we employed an alternative ON switch utilizing another input protein, S15, and confirmed that the OFF (OFF-Kt or OFF-dKt) and ON (ON-Fr15 or ON-dFr15) switches specifically respond to the corresponding inputs, L7Ae and S15, respectively ( Fig. 6b ). 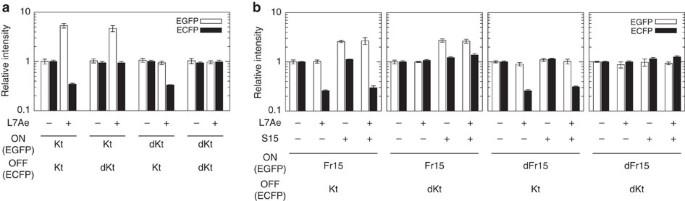Figure 6: Simultaneous and symmetrical control of two outputs in a cell by using ON and OFF switches. (a) The behaviour of ON and OFF switches responsive to a single input (L7Ae). Two reporter proteins, EGFP and enhanced cyan fluorescent protein (ECFP), were produced from ON and OFF switches, respectively. Two OUTPUT plasmids expressing either an ON or an OFF switch (100 ng each) were transfected into HeLa cells together with 20 ng of cognate and 480 ng of noncognate INPUT plasmids. The fluorescent signals were normalized by those of the switches containing Kt in the absence of L7Ae. (b) Control of two switches under two input proteins. Kt or dKt in ON switches were replaced with Fr15 or dFr15 (defective Fr15). Two OUTPUT plasmids were transfected together with L7Ae- (20 ng) and/or S15- (480 ng) expressing plasmids. In this experiment, a viral nucleocapside protein was used as a noncognate RNA-binding protein. The fluorescent signals were normalized by those detected in the absence of both L7Ae and S15. Transfected cells were analysed using FACSAria. Bars and error bars represent the mean and s.d., respectively, of three replicates. Figure 6: Simultaneous and symmetrical control of two outputs in a cell by using ON and OFF switches. ( a ) The behaviour of ON and OFF switches responsive to a single input (L7Ae). Two reporter proteins, EGFP and enhanced cyan fluorescent protein (ECFP), were produced from ON and OFF switches, respectively. Two OUTPUT plasmids expressing either an ON or an OFF switch (100 ng each) were transfected into HeLa cells together with 20 ng of cognate and 480 ng of noncognate INPUT plasmids. The fluorescent signals were normalized by those of the switches containing Kt in the absence of L7Ae. ( b ) Control of two switches under two input proteins. Kt or dKt in ON switches were replaced with Fr15 or dFr15 (defective Fr15). Two OUTPUT plasmids were transfected together with L7Ae- (20 ng) and/or S15- (480 ng) expressing plasmids. In this experiment, a viral nucleocapside protein was used as a noncognate RNA-binding protein. The fluorescent signals were normalized by those detected in the absence of both L7Ae and S15. Transfected cells were analysed using FACSAria. Bars and error bars represent the mean and s.d., respectively, of three replicates. Full size image Signal inversion is one of the most fundamental processes in a circuit. Similar to electrical engineering, complicated biological circuits utilize many signal inversions [21] , [22] , [23] . In many instances, synthetic biologists have employed trans -acting effector and sensor pairs as inverter modules ( Supplementary Fig. S1a,b ). This approach requires at least one unique regulatory pair for every inversion, and performing the inversion in a cell requires a highly independent pair to avoid cross-talk between signalling circuits, which would likely represent a major problem. To avoid this potential pitfall, recent efforts have been made to generate numerous orthogonal regulatory pairs [24] . Unfortunately, although many orthogonal pairs could potentially be developed to generate new sets of trans -acting effectors and sensors, the number of such sets is finite. In contrast, the ON switches produced by the cis -acting module allow the input molecules to directly determine the output protein levels in the absence of additional factors. Moreover, the cis -acting module is advantageous when compared with trans -acting modules because it will likely enable the inversion of multiple signals with similar efficiency ( Supplementary Fig. S1c ). The dynamic range of each inverted switch will differ and will be determined by the nature of the corresponding module in the case of trans -acting modules ( Supplementary Fig. S1b ). In this study, we developed a cis -acting inverter module that is 2.1 kb in length. This relatively large module might cause a problem for handling or integrating the module into the genome of target cells in the future applications. We succeeded in replacing the original β-globin intron (476 nucleotides) with the shorter chimeric intron (133 nucleotides) without sacrificing the efficiency of the inverter module ( Supplementary Fig. S3b ). Moreover, the module with a shortened distance between PTC and the splice site of the intron (320 nucleotides) maintained the efficiency ( Supplementary Fig. S3a ). These results indicate that more compact modules could be designed and constructed by using these elements. Furthermore, a module containing another bait ORF (the part of EGFP gene) functioned as an inverter ( Supplementary Fig. S11 ). Thus, we assume that a bait ORF is likely to be replaced with desired protein-coding sequences. Our module could be employed to develop new ON switches from available translational OFF switches in which the 5′-UTRs of the mRNAs respond to a variety of input molecules, including small molecules, RNA and proteins, in eukaryotic cells [10] , [11] , [12] , [13] , [14] , [15] . In addition, it should also be possible for our module to invert ON switches [8] to OFF switches, because the IRES-driven production of an output protein from the inverted switches is inversely related to the activity of the cap-dependent translation of the bait ORF that corresponds to the output of the parental switches. Finally, the method that we have shown in the present study enables the detection of proteins in the cytoplasm, whereas another synthetic RNA device has been reported that can detect nuclear protein expression to control genetic circuits by employing alternative splicing [11] . Thus, the two types of switches are now available that work in either the nucleus or the cytoplasm. Plasmid constructions We used p1-box C/D-EGFP and p1-box C/D mut-EGFP [10] as parental OFF-switch mRNAs responsive to Archaeoglobus fulgidus L7Ae (OFF-Kt) and its negative control (OFF-dKt), respectively. The Fr15 RNA motif [19] , to which Bacillus stearothermophilus S15 (BS15) binds, was amplified from the DNA template 5′-GGGATGTCAGGTGCAGGCCAGACCGAAGTCCTCTCCTGCCCTCAAGTCTTTCGACC ATCCCTATAGTGAGTCGTATTAGC-3′ by PCR using the primer set 5′-GCTAATCCATGGGATCCTCGGTCGAAAGACTTGAGGGC-3′/5′-CCCAGATCTCGTCAGGTGCAGGCCAGAC-3′, digested with Bam HI and Bgl II, and cloned into the Bgl II– Bam HI site of p1-box C/D-EGFP to construct OFF-Fr15. A negative control plasmid for the switch responsive to BS15 was constructed in the same way, except that a different DNA template (5′-GGGATGTGAGGTGCAGGCCGGACCGAAGTCCTCTCCTGCCCTCAAGTCTTTCGACCATC CCTATAGTGAGTCGTATTAGC-3′) was used. The switch-inverting module composed of the Renilla luciferase ORF containing nonsense mutations, an intron from the β-globin gene and IRES2. pLP1 (Invitrogen, Carlsbad, CA) was digested with Bam HI and Bgl II, and a DNA fragment containing the β-globin intron was inserted into the Bam HI site of pIRES2-EGFP (Clontech Laboratories, Mountain View, CA). The Bam HI site of the resulting plasmid was removed by digestion with Bam HI, followed by Klenow fragment treatment (Takara Bio, Otsu, Japan) and self-ligation to construct pdBIntIRES2-EGFP. The 5′-UTR of p1-box C/D-EGFP was obtained by digestion with Nhe I and Nco I, purified by PAGE and then inserted into the Nhe I– Nco I site of pGL4.73 (Promega, Madison, WI). Both W153 and W156 of Renilla luciferase were replaced with a stop codon by PCR mutagenesis using the following primer set: 5′-GTGACCTGACATCGAGGAGGATA-3′ and 5′-TCGTCTCAGGACTCGATCACGTCC-3′. The Nhe I– Nae I fragments from the resulting and the parental plasmid were inserted into the Nhe I– Sma I site of pdBIntIRES2-EGFP to generate a plasmid that expresses ON-Kt and ONn-Kt, respectively. Their Age I– Bsp 1407I fragments were used to invert other OFF switches. IRES and Bim-EL were amplified from pIRES2-EGFP and pBim [12] by PCR using a primer set: 5′-CGCAAATGGGCGGTAGGCGTG-3′/5′-CATGGTTGTGGCCATATTATCATCG-3′ and 5′-CGATGATAATATGGCCACAACCATGGCAAAGCAACCTTCTGATG-3′/5′-GCCCCGCAGAAGGTCTAGAATCAATGCATTCTCCACACCAG-3′, respectively. These fragments were concatenated by PCR again using a primer set: 5′-CGCAAATGGGCGGTAGGCGTG-3′/5′-AAGCTTGCGGCCGCCCCGCAGAAGGTCTAGA-3′, digested with Hin dIII and Not I and inserted into Hin dIII– Not I site of pON-Kt/dKt to generate pON-Kt/dKt-B, respectively. INPUT plasmids express RNA-binding proteins fused to a One-STrEP-tag (IBA, Göttingen, Germany) at the N-terminus and to a myc-tag and His-tag at the C-terminus, together with IRES-driven DsRed-Express under control of the cytomegalovirus promoter. Briefly, the RNA-binding proteins were cloned into pcDNA5/FRT/TO (Invitrogen) containing the expression cassette from pIRES2-DsRed-Express (Clontech Laboratories). pIRES2-DsRed-Express was digested with Bam HI and Not I, and the fragment containing the IRES2-driven DsRed-Express expression cassette was cloned into the Bam HI– Not I site of pcDNA5/FRT/TO (Invitrogen). The Hin dIII-digested fragment from p4LambdaN22-3mEGFP-M9 (ref. 25 ) was inserted into the resulting expression vector. Then, four Lambda N22 peptide repeats were replaced by the RNA-binding proteins that were amplified by PCR and fused to the peptide tags. The ORFs of A. fulgidus L7Ae, the bacteriophage MS2 coat protein, B. stearothermophilus S15 and HIV nucleocapsid protein were amplified using the primer sets 5′-GAATCCATGGGATCCATGTACGTGAGATTTGAGGTTC-3′/5′-CACCAGATCTCTTCTGAAGGCCTTTAATCTTCTC-3′, 5′-CACCATGGGATCCGCTTCTAACTTTACTCAGTTCGTTCTC-3′/5′-TATGAGATCTGTAGATGCCGGAGTTGGC-3′, 5′-GACACCATGGGATCCGCATTGACGCAAGAGCG-3′/5′-TATGAGATCTTCGACGTAATCCAAGTTTCTCAAC-3′ and 5′-GCTACCATGGGATCCATACAGAAAGGCAATTTTAGGAAC-3′/5′-CCCTAGATCTATTAGCCTGTCTCTCAGTACAATCT-3′, from the pL7Ae [10] , MS2-EGFP [26] plasmids and a newly synthesized plasmid based on a previous study [27] , and pLP2 (Invitrogen), respectively. For apoptosis assay, DsRed-Express in INPUT plasmids was replaced by EGFP of pIRES2-EGFP using Avr II and Not I restriction sites. Cell culture and transfection of plasmids HeLa cells were cultured at 37 °C and 5% CO 2 in DMEM (GIBCO, Carlsbad, CA) containing 10% fetal bovine serum (Nichirei Biosciences, Tokyo, Japan) and a 1% antibiotic–antimycotic solution (Sigma-Aldrich, St Louis, MO). A total of 5 × 10 4 cells were seeded in 24-well plates, and after 24 h, 70–90% confluent cells were transiently transfected with 100 mg of an OUTPUT plasmid and 500 mg of the INPUT plasmids using 1 μl of Lipofectamine 2000 (Invitrogen), following the manufacturer’s instructions. The medium was changed 4 h after transfection. Fluorescent microscopy analysis Fluorescent images were captured 24 h after transfection using a fluorescent microscope system (IX81; Olympus, Tokyo, Japan) with NIBA and WIGA mirror units (Olympus) for EGFP and DsRed-Express detection, respectively. The acquired EGFP images were contrast-enhanced using ImageJ software (NIH, Bethesda, MD). Flow-cytometry analysis Twenty-four hours after transfection, the cells were washed with PBS and incubated in 100 μl of 0.25% Trypsin-EDTA (GIBCO) for 2 min at 37 °C. After addition of 100 μl of medium, the cells were passed through a 35 μm strainer (BD Biosciences, San Jose, CA) and then analysed with a FACSAria cell sorter (BD Biosciences) or BD Accuri (BD Biosciences). A 488-nm semiconductor laser and 530/30 and 695/40 nm filters were used for EGFP and DsRed-Express detection, respectively. A 408-nm semiconductor laser for excitation and a 450/40-nm filter for emission were used to measure the fluorescence of enhanced cyan fluorescent protein and Pacific Blue. For the analysis using BD Accuri, a 585/40-nm filter was used to detect DsRed-Express. In reporter assays, dead cells were gated out based on their forward and side scatter properties. Fluorescent signal compensation was not required for the ranges of fluorescence intensity observed in experiments using FACSAria. In the analysis using BD Accuri, fluorescent signals were compensated based on a compensation matrix, coefficients of which were determined by a linear fitting of signals from cells expressing either EGFP or DsRed-Express. To evaluate the behaviour of the switches, geometric mean of the ratio between EGFP and DsRed-Express fluorescence was calculated from the transfected cells, which showed higher signals than the autofluorescence. To assess the analytical procedure, we compared representative values derived from different methods. Details are available in Supplementary Methods . Isolation of total RNA and complementary DNA synthesis Twenty-four hours after transfection, the cells were washed with chilled PBS. Then, total RNA was isolated using the RNAqueous-4PCR Kit (Ambion, Carlsbad, CA) following the manufacturer’s instructions. RNA was extracted using 350 μl of Lysis/Binding Solution and eluted in 50 μl of Milli-Q water twice. Contaminating DNA was removed using the TURBO DNA-free Kit (Ambion). cDNA was synthesized from 200 ng of the total extracted RNA using High-Capacity cDNA Reverse Transcription Kits (Applied Biosystems, Carlsbad, CA). The resulting cDNA solutions were diluted 10-fold, and 5 μl aliquots were subjected to quantitative RT–PCR analysis. Quantitative RT–PCR analysis Quantitative RT–PCR analysis was carried out using LightCycler 480 SYBR Green I Master kits (Roche, Basel, Switzerland) and LightCycler 480 instruments (Roche). The reaction mixtures contained the primer set 5′-GAAGCGCGATCACATGGT-3′/5′-CCATGCCGAGAGTGATCC-3′ or 5′-GGCTACCCGTGATATTGCTG-3′/5′-GCGATACCGTAAAGCACGA-3′ at a final concentration of 500 nM for the purpose of measuring the level of EGFP- (switch mRNAs) or neomycin-resistant gene mRNA (control for normalization), respectively. A series of 10-fold dilutions of the output plasmid (50 fg–5 ng) was used as a standard of measurement. The relative amounts of the switch mRNAs were determined based on those of the neomycin-resistant gene mRNA expressed from the same output plasmid. The average and s.d. from triplicate experiments are presented. RNA interference knockdown A total of 2.5 × 10 4 cells were seeded in 24-well plates, and after 24 h, cells were transfected with 20 pmol of siRNA using 1 μl of StemFect RNA transfection kit (Stemgent, Cambridge, MA) according to the manufacturer’s instruction. The medium was changed 4 h after transfection. After 48 h, a set of plasmids were transfected as described above. Then, after 24 h, the cells were subjected to flow-cytometry analysis using BD Accuri. According to the previous studies [28] , the sequences of siRNA used in this experiment were as follows: 5′-GUGUAUGUGCGCCAAAGUATT-3′/5′-UACUUUGGCGCACAUACACTT-3′ (SMG1), 5′-GAUGCAGUUCCGCUCCAUUTT-3′/5′-AAUGGAGCGGAACUGCAUCTT-3′ (UPF1), 5′-CAACAGCCCUUCCAGAAUCTT-3′/5′-GAUUCUGGAAGGGCUGUUGTT-3′ (UPF2) and 5′-UUCUCCGAACGUGUCACGUTT-3′/5′-ACGUGACACGUUCGGAGAATT-3′ (non-silencing negative control). Western blotting analysis Transfection experiments were performed in four times larger scale in six-well plates compared with that in 24-well plates. After 24 h (plasmid transfection) or 48 h (RNA interference knockdown), transfected cells were washed twice with 2 ml of PBS and extracted in 0.3 ml of RIPA buffer. Concentration of total protein was measured by BCA Protein assay (Thermo, Rockford, IL). Samples (10 μg) were subjected to SDS–PAGE, transferred into a polyvinylidene difluoride membrane using iBlot (Invitrogen) following the manufacturer’s instruction and probed with indicated antibodies followed by horseradish peroxidase-conjugated secondary antibodies. SMG1 and RENT1 antibody (Bethyl Laboratories, Montgomery, TX), and UPF2 rabbit monoclonal antibody (D3B10; Cell Signaling Laboratory, Danvers, MA) were used at 1000-fold dilution. GAPDH antibody (Santa Cruz Biotechnology, Santa Cruz, CA) and anti-c-Myc mouse monoclonal antibody (9E10; Calbiochem, Darmstadt, Germany) were used at 100-fold and 200-fold dilution, respectively. The blots were detected with Immobilon Western Chemiluminescent horseradish peroxidase substrate (Millipore, Billerica, MA) and ImageQuant LAS 4000 (GE Healthcare, Piscataway, NJ). Apoptosis assay Alternative INPUT plasmids, which express EGFP instead of DsRed-Express, were used in this experiment. Twenty-four hours after transfection of the plasmids, the cells and medium were collected, stained with annexin V, Pacific Blue conjugates (Invitrogen) according to the manufacturer’s instruction and analysed using a FACSAria cell sorter. Untransfected cells were gated out based on EGFP fluorescence. The average and s.d. from two independent experiments are presented. How to cite this article: Endo, K. et al . A versatile cis -acting inverter module for synthetic translational switches. Nat. Commun. 4:2393 doi: 10.1038/ncomms3393 (2013).